Cambrian lobopodians and extant onychophorans provide new insights into early cephalization in Panarthropoda Cambrian lobopodians are important for understanding the evolution of arthropods, but despite their soft-bodied preservation, the organization of the cephalic region remains obscure. Here we describe new material of the early Cambrian lobopodian Onychodictyon ferox from southern China, which reveals hitherto unknown head structures. These include a proboscis with a terminal mouth, an anterior arcuate sclerite, a pair of ocellus-like eyes and branched, antenniform appendages associated with this ocular segment. These findings, combined with a comparison with other lobopodians, suggest that the head of the last common ancestor of fossil lobopodians and extant panarthropods comprized a single ocular segment with a proboscis and terminal mouth. The lack of specialized mouthparts in O. ferox and the involvement of non-homologous mouthparts in onychophorans, tardigrades and arthropods argue against a common origin of definitive mouth openings among panarthropods, whereas the embryonic stomodaeum might well be homologous at least in Onychophora and Arthropoda. The great diversity of arthropod body plans is reflected by the manifold architecture of their heads. This diversity might have its origins in the early Cambrian or even Pre-Cambrian periods [1] , [2] , [3] , when the three major groups of Panarthropoda diverged: Onychophora (velvet worms), Tardigrada (water bears) and Arthropoda (spiders, centipedes, insects and alike). The trunk anatomy of the last common ancestor of panarthropods most likely resembled that of fossil lobopodians, which share with extant onychophorans and tardigrades a homonomous body segmentation, a soft cuticle without an exoskeleton, and unjointed limbs called lobopods [4] , [5] , [6] , [7] . Despite these similarities, the structure and composition of the head among the extant panarthropods are so diverse that it is hard to believe that their heads have a common evolutionary origin. A closer look at the head morphology in fossil lobopodians, thus, might help to unravel the early steps in the diversification of panarthropod heads. So far, however, little is known about the head structure in these ancient animals, mostly because of an incomplete preservation of their anterior ends [8] , [9] , [10] , [11] , [12] , [13] , [14] . We therefore analysed exceptionally preserved specimens of the lower Cambrian lobopodian Onychodictyon ferox [15] and compared its head anatomy with that in other lobopodians and extant panarthropods. In addition, we examined mouth development in the recent onychophoran Euperipatoides rowelli , which sheds new light on the homology of mouth openings among panarthropods. Overview The taxon Lobopodia established by Snodgrass [16] most likely comprizes a non-monophyletic assemblage [1] , [4] , [12] , [13] of stem-group representatives of Panarthropoda, Onychophora, Tardigrada and Arthropoda. The exact phylogenetic position of O. ferox among non-cycloneuralian ecdysozoans is unresolved [11] , [12] , [13] , [14] , [17] . Emended diagnosis of O. ferox Armoured lobopodian; anterior end (head region) characterized by a bulbous proboscis, a pair of lateral eyes associated with a pair of dorsolateral, feather-like antenniform appendages and an unpaired arcuate sclerite; mouth terminal, succeeded by a buccal tube leading into a pharyngeal bulb followed by a through-gut; trunk consisting of homonomous segments bearing 12 pairs of unjointed walking limbs (lobopods) with paired claws and 10 pairs of dorsal sclerotized plates; trunk posteriorly merges with last leg pair; body wall and all appendages densely annulated and covered by a thin cuticle (no exoskeleton); and long, slender papillae present on trunk, legs and antenniform appendages. Trunk anatomy in O. ferox The trunk anatomy of the new material of O. ferox (186 specimens; Supplementary Table S1 ) corresponds with earlier descriptions [15] , [18] because complete specimens show 10 pairs of sclerotized dorsal plates with thorn-like spines and 12 pairs of annulated lobopods, bearing longitudinal rows of papillae and a pair of sickle-like claws ( Figs 1 and 2a–c ). The bases of the two posterior-most pairs of limbs are in close proximity, and there is no posterior continuation of the trunk. Numerous finger-like papillae, typically with only the imprints of their bases preserved, are arranged in longitudinal rows along the trunk, and ventrally additional rows of more prominent papillae point downwards ( Fig. 2a ). In contrast to previous descriptions [15] , [18] of a ‘short, rounded’ head [15] , our specimens show a more complex anatomy of the anterior end than hitherto realized ( Figs 1 and 2a–h ; Supplementary Figs S1–S6 ). 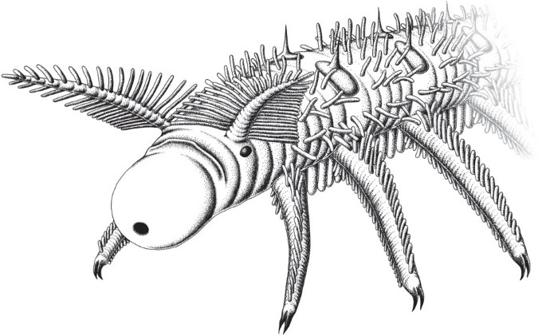Figure 1: Anterior body region of the lobopodianO. ferox. Amongst the most conspicuous structures are the feathery, antenniform appendages, the proboscis with a terminal mouth and the ocellus-like eye at the basis of each antenniform appendage. Figure 1: Anterior body region of the lobopodian O. ferox . Amongst the most conspicuous structures are the feathery, antenniform appendages, the proboscis with a terminal mouth and the ocellus-like eye at the basis of each antenniform appendage. 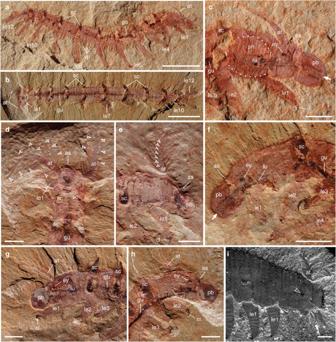Figure 2: Anatomy of the lobopodiansO. feroxandA. pedunculata. (a–h)O. ferox. (a) Laterally compressed specimen ELEL-SJ101888A; anterior is right. (b) Dorsoventrally compressed specimen ELEL-EJ100329A; anterior is left. (c) Close-up of anterior end inashowing head structures and outline of bulbous pharynx (dotted lines). Arrow points to mouth. (d) Close-up of anterior end inbshowing a pair of branched antenniform appendages (branches indicated by arrowheads). (e) Specimen ELEL-SJ102011A showing left antenniform appendage with branches. Note annulations of antenniform appendage (arrowheads) and claws on first walking lobopod. (f) Specimen ELEL-SJ100307B showing an eye with a lens-like structure. Arrow indicates mouth. (g,h) Specimens ELEL-SJ100635 and ELEL-SJ100546A showing anterior anatomy, notably proboscis, eye and branched antenniform appendages. (i) Anterior end ofA. pedunculata. Note branched antenniform appendages, eye-like structure (arrowhead) and putative proboscis delineated from the rest of the body. as, arcuate sclerite; at, antenniform appendage; bt, buccal tube; cl, claw; ey, eye; gu, gut; le1–le12, walking lobopods 1–12; lu, pharyngeal lumen; pb, proboscis; ph, pharynx; sc, sclerotized plate; vp, ventral papillae. Scale bars, 1 cm inaandb; 2 mm inc–i. Full size image Figure 2: Anatomy of the lobopodians O. ferox and A. pedunculata . ( a – h ) O. ferox . ( a ) Laterally compressed specimen ELEL-SJ101888A; anterior is right. ( b ) Dorsoventrally compressed specimen ELEL-EJ100329A; anterior is left. ( c ) Close-up of anterior end in a showing head structures and outline of bulbous pharynx (dotted lines). Arrow points to mouth. ( d ) Close-up of anterior end in b showing a pair of branched antenniform appendages (branches indicated by arrowheads). ( e ) Specimen ELEL-SJ102011A showing left antenniform appendage with branches. Note annulations of antenniform appendage (arrowheads) and claws on first walking lobopod. ( f ) Specimen ELEL-SJ100307B showing an eye with a lens-like structure. Arrow indicates mouth. ( g , h ) Specimens ELEL-SJ100635 and ELEL-SJ100546A showing anterior anatomy, notably proboscis, eye and branched antenniform appendages. ( i ) Anterior end of A. pedunculata . Note branched antenniform appendages, eye-like structure (arrowhead) and putative proboscis delineated from the rest of the body. as, arcuate sclerite; at, antenniform appendage; bt, buccal tube; cl, claw; ey, eye; gu, gut; le1–le12, walking lobopods 1–12; lu, pharyngeal lumen; pb, proboscis; ph, pharynx; sc, sclerotized plate; vp, ventral papillae. Scale bars, 1 cm in a and b ; 2 mm in c – i . Full size image Head anatomy in O. ferox The new material reveals that the anterior-most portion of the head comprizes a bulbous proboscis, delineated from the rest of the body by a circumferential constriction. A terminal mouth extends into a straight buccal tube ( Figs 1 and 2c ; Supplementary Figs S1–S3 ). In laterally preserved specimens, the anterior end can be seen to be bent slightly ventrally ( Fig. 2a ; Supplementary Figs S1–S4 ). This accounts for why the proboscis is not seen in specimens preserved in other aspects ( Fig. 2b ; Supplementary Table S1 ) and, hence, remained undetected in previous studies [15] , [18] . The proboscis is succeeded by the first body segment, which bears a pair of eyes and antenniform appendages. The eyes are represented by carbonaceous remains of simple, ocellus-like structures situated dorsolaterally on the head. Adjacent to these is a pair of annulated antenniform appendages with numerous branches ( Figs 1 and 2c–h ; Supplementary Figs S1–S5 ). Another prominent feature of the head is a structure posterior to the proboscis, belonging to the first body segment and referred to as the ‘arcuate sclerite’ ( Figs 1 and 2c–f ; Supplementary Figs S1, S6 ). In contrast to the first and the remaining body segments, sclerotized structures of any sort are not evident in the second segment, which bears the first pair of walking lobopods ( Figs. 1 and 2c–h ; Supplementary Figs S1–S4 ). A conspicuous feature of this second segment is an internal bulbous structure with an expanded lumen and dark contents, which anteriorly joins the buccal tube and posteriorly the alimentary canal ( Fig. 2c ; Supplementary Fig. S1 ). We regard this bulbous structure as a suctorial pharynx on account of its resemblance in position and shape to the pharynx of extant tardigrades and onychophorans [19] , [20] ( Supplementary Fig. S7 ). Mouth development in Onychophora During embryonic development of the onychophoran E. rowelli , three consecutive mouth openings arise ventrally ( Fig. 3a–f ). The first mouth occurs anteriorly in the embryonic disc, when the lateral lips of the blastopore close by amphystomy ( Fig. 3a ). During further development, the ectoderm surrounding this first mouth opening invaginates and forms the second mouth, that is, the stomodaeum, the walls of which eventually give rise to the adult pharynx [21] , [22] , [23] ( Fig. 3b ; Supplementary Fig. S7 ). During stomodaeum development, the orifice of the first (blastoporal) mouth is internalized and, thus, corresponds to the posterior border of the presumptive pharynx ( Fig. 3a ). The stomodaeum is initially located at the border between the first and second body segments ( Fig. 3b ). As development proceeds, large ectodermal areas surrounding the stomodaeum sink into the embryo—a process by which the stomodaeum and the anlagen of jaws and tongue are incorporated into the newly formed mouth cavity ( Fig. 3c–f ). This cavity persists in adults and opens to the exterior via the definitive (third) mouth opening ( Fig. 3e ; Supplementary Fig. S7 ). During ontogeny, this mouth opening is formed by an accumulation of lips that originate from the antennal, jaw and slime papilla segments and aggregate around the mouth ( Fig. 3c–e ). At the end of embryogenesis, the stomodaeum disappears completely within the definitive mouth cavity, and its initial opening corresponds to the anterior border of the presumptive pharynx ( Fig. 3d–f ; Supplementary Fig. S7 ). 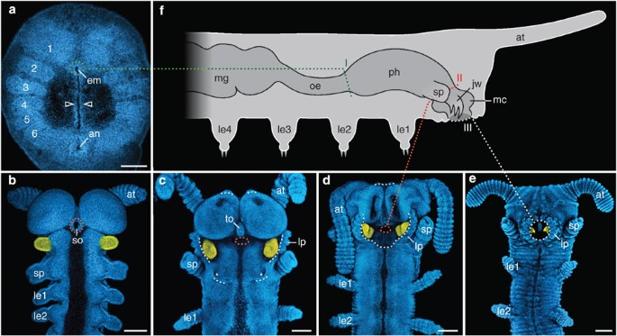Figure 3: Mouth development in the onychophoranE. rowelli. Note that three consecutive mouth openings arise during onychophoran ontogeny (indicated by green, red and white dotted lines, respectively). (a–e) Confocal micrographs of embryos at subsequent developmental stages52in ventral view, labelled with the DNA-marker Hoechst as described previously60. Anterior is up. Presumptive jaws are coloured artificially in yellow. (a) Embryonic disc of a late stage 1 embryo. Note the first embryonic mouth (em) arising at the anterior end of the slit-like blastopore. Developing segments are numbered. Arrowheads point to closing blastoporal lips. (b) Anterior end of an early stage 4 embryo. Note the position of the stomodaeum (second mouth) at the posterior border of the antennal segment. (c) Anterior end of a late stage 4 embryo. Note the beginning formation of lips that originate from three different segments (white dotted lines). Asterisks indicate openings of presumptive salivary glands. (d) Anterior end of a stage 5 embryo showing the formation of the definitive (third) mouth. Note that the stomodaeum and the anlagen of jaws and tongue are incorporated into the mouth cavity. (e) Anterior end of a stage 7 embryo. Mouth development is completed and lips surround the circular mouth opening. (f) Diagram of an adult onychophoran illustrating regions of digestive tract that correspond to the three consecutive embryonic mouth openings (dotted lines with Roman numerals I–III). Dorsal is up, anterior is right. an, developing anus; at, antenna; em, first embryonic mouth (derivative of the blastopore); jw, jaw; le1–le4, legs 1–4; lp, developing lips; mc, mouth cavity; mg, midgut; oe, oesophagus; ph, pharynx; so, stomodaeum; sp, slime papilla; to, presumptive tongue. Scale bars, 200 μm ina–e. Figure 3: Mouth development in the onychophoran E. rowelli . Note that three consecutive mouth openings arise during onychophoran ontogeny (indicated by green, red and white dotted lines, respectively). ( a – e ) Confocal micrographs of embryos at subsequent developmental stages [52] in ventral view, labelled with the DNA-marker Hoechst as described previously [60] . Anterior is up. Presumptive jaws are coloured artificially in yellow. ( a ) Embryonic disc of a late stage 1 embryo. Note the first embryonic mouth (em) arising at the anterior end of the slit-like blastopore. Developing segments are numbered. Arrowheads point to closing blastoporal lips. ( b ) Anterior end of an early stage 4 embryo. Note the position of the stomodaeum (second mouth) at the posterior border of the antennal segment. ( c ) Anterior end of a late stage 4 embryo. Note the beginning formation of lips that originate from three different segments (white dotted lines). Asterisks indicate openings of presumptive salivary glands. ( d ) Anterior end of a stage 5 embryo showing the formation of the definitive (third) mouth. Note that the stomodaeum and the anlagen of jaws and tongue are incorporated into the mouth cavity. ( e ) Anterior end of a stage 7 embryo. Mouth development is completed and lips surround the circular mouth opening. ( f ) Diagram of an adult onychophoran illustrating regions of digestive tract that correspond to the three consecutive embryonic mouth openings (dotted lines with Roman numerals I–III). Dorsal is up, anterior is right. an, developing anus; at, antenna; em, first embryonic mouth (derivative of the blastopore); jw, jaw; le1–le4, legs 1–4; lp, developing lips; mc, mouth cavity; mg, midgut; oe, oesophagus; ph, pharynx; so, stomodaeum; sp, slime papilla; to, presumptive tongue. Scale bars, 200 μm in a – e . Full size image According to our findings, the paired antenniform appendages of O. ferox , which are associated with the ocular segment, differ from walking lobopods in three respects: (i) they lack terminal claws, (ii) they bear on either side slender projections decreasing in length distally and (iii) they have bases that insert dorsolaterally on the ocular segment rather than ventrolaterally. Before this discovery, the identity of the anterior-most pair of appendages in O. ferox has remained controversial [15] , [17] , [18] , [24] . An original identification of putative antennae [15] was then rejected [11] , [18] , [25] , but subsequently gained some support [17] . In addition, the anterior-most pair of clawed lobopods were reinterpreted as a pair of modified cephalic appendages [18] , [24] . Our material, however, shows that the first pair of lobopods do not differ from succeeding pairs and so form a homonomous series of ventral annulated limbs equipped with longitudinal rows of papillae and terminal claws. The pair of antenniform cephalic appendages identified here, thus, lie in front of the first pair of clawed lobopods. Given their location on the ocular segment, we suggest that these appendages are homologous to the branched anterior appendages of Aysheaia pedunculata [9] ( Fig. 2i ), the first pair of unbranched antenniform appendages of Antennacanthopodia gracilis [26] , and to the antennae of extant onychophorans [23] . In contrast, the homology of these appendages with segmental limbs of crown-group arthropods is more difficult to establish because of many divergent views on the composition and evolution of the arthropod heads [5] , [27] , [28] , [29] , [30] , [31] , [32] , [33] , [34] , [35] , [36] . The equivalents of the first pair of appendages might have been lost in extant arthropods because the anterior-most segment in these animals does not show typical modified limbs [33] , [34] , [37] . Alternatively, the so-called ‘labrum’ might be a possible homologue or remnant of this pair of limbs [32] , [38] , [39] . However, this view depends on whether the labrum belongs to the first/ocular segment [32] , [33] , or to the third/intercalary segment [27] , [28] , or whether it is an independent morphological structure/unit/segment anterior to the eye region [29] , [40] . Thus, even among the insect species studied, the segmental identity of the labrum is uncertain, not to mention the homology of various structures referred to as a ‘labrum’ throughout the four major arthropod groups (chelicerates, myriapods, crustaceans and insects). In fact, some authors suggest that a true labrum only exists in the in-group crustacean taxon Labrophora [30] , [31] . We therefore caution against an uncritical homologization of structures identified as a ‘labrum’ among crown-group arthropods. Likewise, the homology of various cephalic appendages across stem-group and crown-group arthropods is controversial. Major inconsistency concerns the so-called ‘great appendages’, which have been assigned to the first [32] , second [5] , [33] , [34] , [35] or third cephalic segments [36] . One of the reasons for the lack of consensus might be insufficient information on head development from fossils. As is well known from work on living arthropods, segmental identities of anterior appendages are difficult to establish without analysing gene-expression patterns and details of embryology [41] , [42] . It seems therefore premature to speculate on the homology of ‘great appendages’ across panarthropods with complex, composite heads. In contrast, the early cephalization events of stem-group panarthropods might be easier to understand, given the low complexity of their ‘heads’. According to our findings, the anterior-most, antenniform appendages of O. ferox are homologous to the antennae of onychophorans [23] , [37] , [38] , [39] . Thus, they can be regarded as ‘primary antennae’, whereas the equivalents of ‘secondary antennae’ (=first antennae of the mandibulate taxa) [33] in O. ferox are unmodified walking limbs. Ocellus-like visual organs similar to those reported here from specimens of O. ferox are found in the coeval lobopodians Miraluolishania haikouensis [43] , Luolishania longicruris [12] and A. gracilis [26] , as well as extant Onychophora [44] . In addition, ocellus-like structures occur in A. pedunculata [9] ( Fig. 2i ) and extant Tardigrada [45] . Evidence from the innervation pattern [44] and opsins [46] in Onychophora suggests that simple, ocellus-like eyes are an ancestral feature of Panarthropoda, whereas compound eyes evolved in the arthropod lineage. This hypothesis receives support from the organization of visual organs in fossil lobopodians, given their non-monophyly and phylogenetic position near the basis of the panarthropod tree [2] , [6] , [12] , [13] . We therefore suggest that the eyes of fossil lobopodians and extant onychophorans are homologous and that ocelli were the only type of visual organs present in their last common ancestor. These visual organs might have persisted as median ocelli in extant arthropods [44] , whereas subsequent multiplication and modification of these structures gave rise to the ommatidia of compound eyes [47] , [48] . The position and near-vertical orientation of the arcuate sclerite in O. ferox suggest that this structure might have served as an attachment site for the proboscis musculature. To date, this sclerite has not been reported from other lobopodians and might represent an apomorphy of O. ferox . Notably, re-examination of the Burgess Shale lobopodian A. pedunculata reveals what may be a bulbous proboscis, delineated by a constriction ( Fig. 2i ; Delle Cave and Simonetta [8] but see Whittington [9] for an opposed view). Taking into account that lobopodians might be a paraphyletic grade [1] , [4] , [6] , [12] , [13] and that A. pedunculata is one of the earliest-branching lobopodians [6] , [12] , we suggest that a non-segmental proboscis with a terminal mouth was present in the last common ancestor of Cambrian lobopodians and extant panarthropods. Whether this structure is homologous to the proboscis of pycnogonids [49] , [50] or to the introvert of some cycloneuralians [51] , which also show a terminal mouth, is open for discussion. Irrespective of this controversy, attempts have been made to homologize the terminal mouth of fossil lobopodians (and cycloneuralians) with the ventral mouth of onychophorans, suggesting that the mouth opening simply migrated to a ventral position in the onychophoran ancestor [38] . However, we have shown here that three different mouth openings arise during onychophoran embryogenesis. This begs the question, which one of these openings can be homologized with the mouths found in other panarthropods. Our data show that the adult onychophoran mouth has a unique ontogenetic fate, as it involves structures that are not found in other animal groups, including lips, tongue and jaws. The lips surrounding the definitive mouth opening originate from the antennal, jaw and slime papilla segments [21] , [22] , [52] . Accordingly, the onychophoran mouth is derived from three anterior-most body segments, whereas the mouth of O. ferox is proboscideal and, therefore, belongs to a pre-antennal, non-segmental body region ( Fig. 4 ). Our data further revealed no appendage-derived mouthparts in O. ferox , whereas onychophorans show a pair of jaws enclosed within a mouth cavity. The jaws are modified limbs of the second body segment, equivalent to the first pair of walking lobopods in O. ferox . On this basis, neither the position (segmental identity) of the adult mouth nor the composition of its cavity indicates homology of mouth apparatuses in onychophorans and O. ferox . 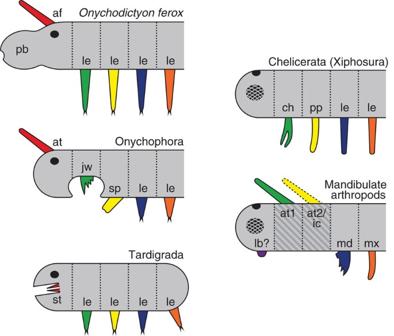Figure 4: Alignment and homology of anterior appendages in the lobopodianO. feroxand among extant panarthropods. Homologous appendages are depicted by corresponding colour. Vertical dotted lines indicate segmental borders. Black and checked ovals represent ocelli and compound eyes, respectively. Alignment of head segments in tardigrades is based on the assumption of serial homology of the stylet with distal leg portions20. Note that segmental identity and homology of the arthropod labrum is discussed controversially30,31,33,40. Dark-grey hatched area in the diagram on mandibulate arthropods indicates segments that do not contribute to adult mouth formation. Note that non-homologous segments and structures are involved in adult mouth apparatuses inO. feroxand different groups of extant panarthropods. af, antenniform appendage; at, antenna; at1, first antenna; at2, second antenna (indicated by a dotted line, as it occurs only in crustaceans); ch, chelicera; ic, intercalary segment (limbless in myriapods and hexapods); jw, jaw; lb, labrum (question mark highlights the uncertain segmental identity and homology of this structure); le, walking limbs/lobopods; md, mandible; mx, maxilla; pb, proboscis; pp, pedipalp; sp, slime papilla; st, stylet. Figure 4: Alignment and homology of anterior appendages in the lobopodian O. ferox and among extant panarthropods. Homologous appendages are depicted by corresponding colour. Vertical dotted lines indicate segmental borders. Black and checked ovals represent ocelli and compound eyes, respectively. Alignment of head segments in tardigrades is based on the assumption of serial homology of the stylet with distal leg portions [20] . Note that segmental identity and homology of the arthropod labrum is discussed controversially [30] , [31] , [33] , [40] . Dark-grey hatched area in the diagram on mandibulate arthropods indicates segments that do not contribute to adult mouth formation. Note that non-homologous segments and structures are involved in adult mouth apparatuses in O. ferox and different groups of extant panarthropods. af, antenniform appendage; at, antenna; at1, first antenna; at2, second antenna (indicated by a dotted line, as it occurs only in crustaceans); ch, chelicera; ic, intercalary segment (limbless in myriapods and hexapods); jw, jaw; lb, labrum (question mark highlights the uncertain segmental identity and homology of this structure); le, walking limbs/lobopods; md, mandible; mx, maxilla; pb, proboscis; pp, pedipalp; sp, slime papilla; st, stylet. Full size image Likewise, owing to the differing positions of the openings and the involvement of different segments, neither the onychophoran nor the O. ferox mouths appear to be homologous with the mouth apparatuses in arthropods and tardigrades ( Fig. 4 ). Various arthropods, including pycnogonids, xiphosurans and entomostracan crustaceans, show no specialized mouth chambers with internalized limbs, whereas in myriapods, hexapods and malacostracan crustaceans, the mouth chamber is formed by several pairs of modified appendages, including the mandibles and the maxillae [33] , [53] (the latter are enclosed within an additional pouch of the head capsule in entognathan hexapods). In tardigrades, the stylet within the buccal tube might be a derivative of the distal limb portions [20] , suggesting that at least one pair of segmental appendages has been incorporated into the tardigrade mouth. We therefore interpret the stylet as a derivative of the first pair of segmental appendages, as there is no evidence of any additional segments in the tardigrade head [54] ( Fig. 4 ). Thus, neither the stylet nor the mandibles or the maxillae belong to segments, which are homologous to the mouth-bearing segments in onychophorans ( Fig. 4 ). Because neither positional nor structural or any other criteria of homology [55] , [56] , [57] are satisfied when comparing the adult mouths in O. ferox , onychophorans and other panarthropods, we suggest that they are not homologous but have divergent evolutionary histories in these animal groups. In contrast, the embryonic stomodaeum might well be homologous at least in Onychophora and Arthropoda. In both taxa, the stomodaeum arises ventrally in the same position, that is, at the border between the first and second body segments ( Supplementary Fig. S8 ), and it gives rise to the corresponding ectodermal foregut structures [21] , [22] , [23] , [58] . Although these correspondences in position and ontogenetic fate support the homology of the stomodaeum, from this stage onwards, the morphogenetic processes of mouth development differ fundamentally between Onychophora and Arthropoda, and even between different arthropod groups [31] , [49] , [53] , [58] . Unlike arthropods, the ontogeny of the adult mouth is conserved in Onychophora and, thus, might recapitulate the evolutionary changes that have taken place in the onychophoran lineage. Contrary to the assumption [38] of a simple ventral migration of the ancestral mouth, we suggest that the mouth cavity of Onychophora has arisen by an invagination of the ectoderm, surrounding an ancestral mouth opening and subsequent incorporation of the second pair of appendages into this cavity. Along with their migration, these appendages were transformed into jaws—a characteristic feature of recent Onychophora. Thus, the definitive mouth of Onychophora is not equivalent to the terminal mouth of Cambrian lobopodians, including O. ferox , and the transformation between the two mouth types can only be understood by finding transitional forms. We therefore believe that the description of detailed head morphologies, as provided herein for O. ferox , from additional lobopodians will shed more light on the evolution of complexity and diversity of mouth apparatuses among extant panarthropods and their Cambrian relatives. Specimens of the lobopodian O. ferox Specimens of O. ferox ( n =186) were collected during 2008–2010 from the Heilinpu (previously Qiongzhusi) Formation (Chengjiang fauna, lower Cambrian, ∼ 520 Ma), Yunnan, southern China. Among these specimens, 84 are preserved with proboscis, 34 with mouth opening, 44 with buccal tube, 36 with pharyngeal bulb, 32 with eyes, 95 with antennal rachis, 65 with antennal branches and 114 with arcuate sclerite ( Supplementary Table. S1 ). All specimens are reposited in the Early Life Evolution Laboratory, China University of Geosciences, Beijing, China. Specimens of E. rowelli and Macrobiotus sp Specimens of E. rowelli were obtained and handled as described previously [59] , [60] . Tardigrades ( Macrobiotus sp.) were obtained from moss samples collected in the Volkspark Großdeuben (Saxony, Germany) and labelled with phalloidin-rhodamine as described for onychophorans [60] . Microscopy and image processing Specimens of the lobopodian O. ferox were photographed using a Canon 5D Mark II digital camera. Details were analysed using a Zeiss Stemi-2000C stereomicroscope (Carl Zeiss MicroImaging GmbH, Jena, Germany), equipped with a Canon 450D digital camera. Specimens of the onychophoran E. rowelli and the tardigrade Macrobiotus sp. were analysed with the confocal laser-scanning microscopes Zeiss LSM 510 META (Carl Zeiss MicroImaging GmbH) and Leica TCS STED (Leica Microsystems, Wetzlar, Germany). Confocal image stacks were processed with Zeiss LSM IMAGE BROWSER v4.0.0.241 (Carl Zeiss MicroImaging GmbH) and Leica AS AF v2.3.5 (Leica Microsystems). Final panels and diagrams were designed with Adobe (San Jose, CA, USA) Photoshop CS4 and Illustrator CS4. How to cite this article: Ou, Q. et al . Cambrian lobopodians and extant onychophorans provide new insights into early cephalization in Panarthropoda. Nat. Commun. 3:1261 doi: 10.1038/ncomms2272 (2012).